Measurement of finite-frequency current statistics in a single-electron transistor Electron transport in nanoscale structures is strongly influenced by the Coulomb interaction that gives rise to correlations in the stream of charges and leaves clear fingerprints in the fluctuations of the electrical current. A complete understanding of the underlying physical processes requires measurements of the electrical fluctuations on all time and frequency scales, but experiments have so far been restricted to fixed frequency ranges, as broadband detection of current fluctuations is an inherently difficult experimental procedure. Here we demonstrate that the electrical fluctuations in a single-electron transistor can be accurately measured on all relevant frequencies using a nearby quantum point contact for on-chip real-time detection of the current pulses in the single-electron device. We have directly measured the frequency-dependent current statistics and, hereby, fully characterized the fundamental tunnelling processes in the single-electron transistor. Our experiment paves the way for future investigations of interaction and coherence-induced correlation effects in quantum transport. The electrical fluctuations in a nanoscale conductor reveal a wealth of information about the physical processes inside the device compared with what is available from a conductance measurement alone [1] , [2] , [3] . Zero-frequency noise measurements are now routinely performed using standard techniques, but, more recently, the detection of higher order current correlation functions, or cumulants, has attracted considerable attention in experimental [4] , [5] , [6] , [7] , [8] , [9] , [10] , [11] , [12] , [13] , [14] , [15] , [16] , [17] , [18] , [19] and theoretical [20] , [21] , [22] studies of charge transport in man-made sub-micron structures. Measurements have, for example, been encouraged by the intriguing connections between current fluctuations and entanglement entropy in solid-state systems [23] , [24] as well as by the possibility to test fluctuation theorems [25] , [26] , [27] at the nanoscale that are now a topic at the forefront of non-equilibrium statistical physics. Experiments on current fluctuations have mainly focused on zero-frequency current correlations [4] , [5] , [6] , [7] , [8] , [9] , [10] , [11] , [12] , [13] , [14] , [15] , [16] whereas measurements of finite-frequency cumulants of the current have remained an outstanding experimental challenge. However, noise detection in a restricted frequency band gives only partial information about correlations and measurements that cover the full frequency range are necessary to access all relevant timescales that characterize the transport process. In a zero-frequency measurement, correlation effects are integrated over a long period of time and important information about characteristic timescales are lost. To observe the dynamical features of the correlations, finite-frequency measurements are required [2] , [3] , [28] , [29] , [30] , [31] , [32] , [33] , [34] . It has even been shown theoretically that the frequency-dependent third cumulant (the skewness) of the current may contain further information about correlations and internal timescales of a system compared with the finite-frequency noise alone, for instance in chaotic cavities [29] and diffusive conductors [30] . 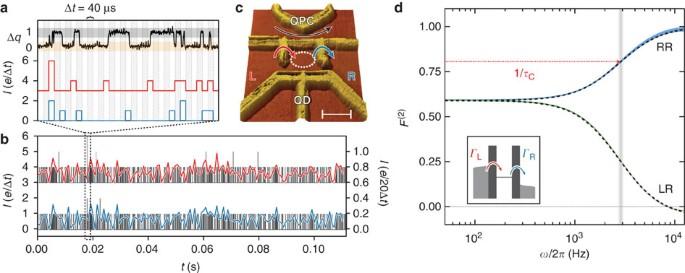Figure 1: SET and finite-frequency noise spectra. (a,b) Fluctuations of the current through the left (red curve) and right (blue curve) tunnelling barriers of the SET. (c) Atomic force microscope topography of the SET consisting of a Coulomb blockade QD coupled through tunnelling barriers to left (L) and right (R) electrodes. The scale bar corresponds to 250 nm. A bias difference between the electrodes drives a stream of electrons through the QD from L to R. An electron entering the QD from L causes a suppression of the current through the nearby QPC until the electron tunnels out of the QD to R. The occupation of the QD (Δq=0, 1) is inferred from the time-dependent current through the QPC (shown with black ina). The corresponding pulse currents through the left (red) and right (blue) barriers are discretized in time steps of Δt=40μs and shown displaced for clarity ina. Inbthe same currents are shown on a much longer timescale and discretized in time steps of Δt(grey spikes) and 20Δt(full lines), respectively. (d) Noise spectrum (blue curve) of the current through the right barrier (RR) and cross-correlations (green curve) between the two currents (LR). The thickness of the lines indicate experimental error estimates. Model calculations (dashed lines) of the spectra are in excellent agreement with the experiment usingΓL=13.23 kHz andΓR=4.81 kHz for the tunnelling rates across the barriers and a detector rate ofΓD=0.3 MHz. The mean dwell time of electrons on the QD isμs and the correlation time isτc=(ΓL+ΓR)−1≃55 μs. The inset shows a schematic model of the charge transport process. Figure 1a–c shows a typical time trace of the currents in our nanoscale single-electron transistor (SET) consisting of a quantum dot (QD) coupled through tunnelling barriers to source and drain electrodes. The QD is operated close to a charge degeneracy point in the Coulomb blockade regime, where only a single extra electron at a time can enter from the source electrode and leave through the drain electrode. The applied voltage bias eV is larger than the electronic temperature k B T which prevents electrons from tunnelling in the opposite direction of the mean current. While a stream of electrons is driven through the QD, a separate current is passed through the nearby quantum point contact (QPC) whose conductance is highly sensitive to the presence of extra electrons (Δ q =0,1) on the QD [35] , [36] . By monitoring the switches of the current through the QPC, we can thus detect, in real-time, single electrons tunnelling through the left (L) and right (R) barriers and thereby determine the corresponding pulse currents I L ( t ) and I R ( t ). The time trace of the currents illustrates the electrical fluctuations of interest here. Figure 1: SET and finite-frequency noise spectra. ( a , b ) Fluctuations of the current through the left (red curve) and right (blue curve) tunnelling barriers of the SET. ( c ) Atomic force microscope topography of the SET consisting of a Coulomb blockade QD coupled through tunnelling barriers to left (L) and right (R) electrodes. The scale bar corresponds to 250 nm. A bias difference between the electrodes drives a stream of electrons through the QD from L to R. An electron entering the QD from L causes a suppression of the current through the nearby QPC until the electron tunnels out of the QD to R. The occupation of the QD (Δ q =0, 1) is inferred from the time-dependent current through the QPC (shown with black in a ). The corresponding pulse currents through the left (red) and right (blue) barriers are discretized in time steps of Δ t =40 μ s and shown displaced for clarity in a . In b the same currents are shown on a much longer timescale and discretized in time steps of Δ t (grey spikes) and 20Δ t (full lines), respectively. ( d ) Noise spectrum (blue curve) of the current through the right barrier (RR) and cross-correlations (green curve) between the two currents (LR). The thickness of the lines indicate experimental error estimates. Model calculations (dashed lines) of the spectra are in excellent agreement with the experiment using Γ L =13.23 kHz and Γ R =4.81 kHz for the tunnelling rates across the barriers and a detector rate of Γ D =0.3 MHz. The mean dwell time of electrons on the QD is μs and the correlation time is τ c =( Γ L + Γ R ) −1 ≃ 55 μs. The inset shows a schematic model of the charge transport process. Full size image We now analyse the current fluctuations obtained from data measured over 24 h during which 300 million electrons passed through the SET. Our high-quality measurements allow us to develop a complete picture of the noise properties of the SET, which not only focuses on the zero-frequency components of the fluctuations, but also contains the full frequency-resolved information about the noise and higher order correlation functions. From the measured finite-frequency noise spectrum, we extract the correlation time of the current fluctuations. The noise spectrum, however, is a one-frequency quantity only which does not reflect correlations between different spectral components of the current. To observe such correlations, we employ bispectral analysis and consider the finite-frequency skewness (or bispectrum) of the current. The skewness shows that the current fluctuations are non-gaussian on all relevant time and frequency scales owing to the non-equilibrium conditions imposed by the applied voltage bias. Our measurements are supported by model calculations that are in excellent agreement with the experimental data. The results presented here provide a fundamental understanding of the electrical fluctuations in SETs that are expected to constitute the basic building blocks of future nanoscale electronics. Noise spectrum The measured noise spectrum for the right tunnelling barrier is presented in Figure 1d . The finite-frequency current-correlation function is defined in terms of the noise power as [1] where , α =L,R, is the Fourier-transformed current and double brackets denote cumulant averaging over many experimental realizations. Figure 1d shows the Fano factor for the right tunnelling barrier with the mean current being constant in the stationary state. The noise is symmetric in frequency, , and results are shown for positive frequencies only. For uncorrelated transport, the noise spectrum would be white, that is, F (2) ( ω )=1 on all frequencies, corresponding to a Poisson process. Our measurements, in contrast, show a clear suppression of fluctuations below the Poisson value at low frequencies. This is due to the strong Coulomb interactions on the QD that introduce correlations in the stream of electrons propagating through the SET: each electron spends a finite time on the QD during which it blocks the next electron entering the QD. The measured noise spectrum has a Lorentzian shape whose width is determined by the inverse dynamical timescale of the correlations. Our measurements of the finite-frequency noise thereby enable a direct observation of the correlation time τ c ≃ 55 μ s of the transport ( Fig. 1d ). To corroborate our experimental results, we calculate the noise spectrum of the schematic model in the inset of Figure 1d . Single electrons tunnel from the left electrode onto the QD at rate Γ L and leave it through the right electrode at rate Γ R . The Fano factor is then [1] where theoretically τ c =(Γ L +Γ R ) −1 is identified as the correlation time. This expression qualitatively explains the measured noise spectrum. Quantitative agreement is obtained by also taking into account the finite detection rate Γ D of the QPC charge-sensing scheme [13] , [37] . The three parameters Γ L , Γ R , and Γ D can be independently extracted from the distribution of waiting times between detected tunnelling events [14] , [38] , [39] . The model calculations (see Methods) are in excellent agreement with measurements over the full range of frequencies, demonstrating the high quality of our experimental data. Cross-correlations Cross-correlations between the left I L ( t ) and the right I R ( t ) currents can also be measured ( Fig. 1d ). For the schematic model, the (cross-correlation) Fano factor reads which in the zero-frequency limit coincides with the noise spectrum, , as a consequence of charge conservation on the QD. The two currents are clearly correlated at frequencies that are lower than the inverse correlation time , but the cross-correlator eventually reaches zero at higher frequencies. Interestingly, the cross-correlations of the detected pulse currents are slightly negative at high frequencies. This is due to the finite resolution of the QPC charge-sensing protocol that is not able to distinguish current pulses that are separated in time by an interval that is shorter than the inverse detector rate . Higher order cumulants We now turn to measurements of higher order finite-frequency cumulants. The m th finite-frequency current correlator corresponding to a time-dependent current I ( t ) is defined as where translational invariance in time implies frequency conservation as indicated by the Dirac delta function δ ( ω ) and S ( m ) ( ω 1 ,..., ω m −1 ) is the polyspectrum [40] , [41] . In the case m =2, the polyspectrum yields the noise power spectrum S (2) ( ω ), whereas the skewness (or bispectrum) is given by m =3 with the corresponding Fano factor F (3) ( ω 1 , ω 2 )= S (3) ( ω 1 , ω 2 )/ e 2 I . We focus here on the frequency-dependent skewness S (3) ( ω 1 , ω 2 ), although our experimental data in principle allows us also to extract cumulants of even higher orders. The measured skewness ( Fig. 2a ), shows a much richer structure and frequency dependence compared with the noise spectrum. The skewness obeys several symmetries following from the definition ( Fig. 2b ). We exploit the mirror symmetry with respect to interchange of frequencies, S (3) ( ω 1 , ω 2 )= S (3) ( ω 2 , ω 1 ), to compare measurement and model calculations: experimental results are presented above the diagonal ( ω 1 = ω 2 ), while model calculations are shown below ( Fig. 2a ). The nonzero bispectrum indicates non-Gaussian statistics on all frequencies and shows strong correlations between different spectral components of the current. Importantly, these correlations are not a consequence of non-linearities in the detection scheme, but are solely due to the physical non-equilibrium conditions imposed by the applied voltage bias. The pulse currents are directly derived from the tunnelling events, and the influence of external noise sources, including the amplification of the QPC current, is thereby explicitly avoided. Intuitively, one would expect the correlations to vanish, if the observation frequency is larger than the average frequency of the transport. Surprisingly, however, a certain degree of correlation persists even if one frequency is large, while the other is kept finite. This is in stark contrast to the second Fano factor F (2) ( ω ) that approaches unity in the high-frequency limit ( Fig. 1d ), corresponding to uncorrelated tunnelling events. 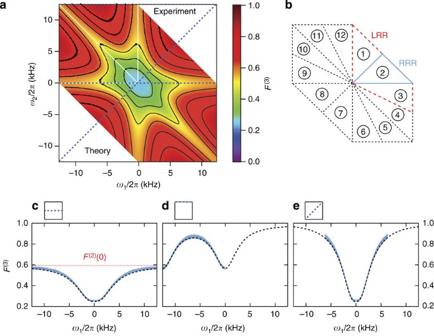Figure 2: Finite-frequency skewness. (a) Experimental results and model calculations of the third Fano factor (the frequency-dependent skewness)F(3)(ω1,ω2)=S(3)(ω1,ω2)/e2I. Experimental results are shown above the diagonal (ω1=ω2) and model calculations below. Contour lines indicateF(3)=0.3, 0.4, 0.5, 0.6, 0.7 and 0.8. The parameters for the model calculations are given in the caption ofFigure 1. (b) Symmetries of the bispectrumF(3)(ω1,ω2). Several important symmetry conditions follow from the definition,40including symmetry with respect to interchange of frequenciesS(3)(ω1,ω2)=S(3)(ω2,ω1). Knowledge of the bispectrum in any of the regions 1–12 is sufficient for a complete description of the bispectrum. We have measured the skewness in region 2 and the cross-bispectrum (Fig. 3) in regions 1–3. (c,d,e) Finite-frequency skewness along the three blue lines ina. Full lines are experimental results, whereas dashed lines show model calculations. The thickness of the full lines indicate the experimental error estimates. The third order Fano factorF(3)(ω1,ω2) approaches the zero-frequency shot noiseF(2)(0) forω2=0 and |ω1| being much larger than the inverse correlation timeas seen inc. Figure 2: Finite-frequency skewness. ( a ) Experimental results and model calculations of the third Fano factor (the frequency-dependent skewness) F (3) ( ω 1 , ω 2 )= S (3) ( ω 1 , ω 2 )/ e 2 I . Experimental results are shown above the diagonal ( ω 1 = ω 2 ) and model calculations below. Contour lines indicate F (3) =0.3, 0.4, 0.5, 0.6, 0.7 and 0.8. The parameters for the model calculations are given in the caption of Figure 1 . ( b ) Symmetries of the bispectrum F (3) ( ω 1 , ω 2 ). Several important symmetry conditions follow from the definition, [40] including symmetry with respect to interchange of frequencies S (3) ( ω 1 , ω 2 )= S (3) ( ω 2 , ω 1 ). Knowledge of the bispectrum in any of the regions 1–12 is sufficient for a complete description of the bispectrum. We have measured the skewness in region 2 and the cross-bispectrum ( Fig. 3 ) in regions 1–3. ( c , d , e ) Finite-frequency skewness along the three blue lines in a . Full lines are experimental results, whereas dashed lines show model calculations. The thickness of the full lines indicate the experimental error estimates. The third order Fano factor F (3) ( ω 1 , ω 2 ) approaches the zero-frequency shot noise F (2) ( 0 ) for ω 2 =0 and | ω 1 | being much larger than the inverse correlation time as seen in c . Full size image For the schematic model in Figure 1d , the finite-frequency skewness reads [32] having defined , and ω 3 = ω 1 + ω 2 . This expression qualitatively explains the measured finite-frequency skewness and shows that the skewness has a complex structure that is not just a simple Lorentzian-shaped function of frequencies. We note that the third Fano factor F (3) ( ω 1 , ω 2 ) reduces to the zero-frequency limit of the noise F (2) (0) in the limit ω 2 =0 and . This is immediately visible in Figure 2c . Again, quantitative agreement is achieved by including the finite detection rate Γ D in the model calculations, as illustrated explicitly in Figure 2c–e . The analytic expression shows that the frequency dependence of the skewness, unlike the auto- and cross-correlation noise spectra, is not only governed by the correlation time τ c . The skewness has an involved frequency dependence, given by several frequency scales, which cannot be deduced from the noise spectrum alone. 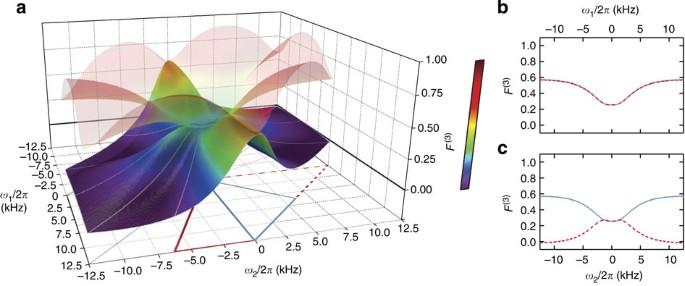Figure 3: Finite-frequency cross-bispectrum. (a) Measurements of the frequency-dependent cross-bispectrum. The cross-bispectrum shows a reduced symmetry compared with the bispectrum and measurements in the regions 1–3 (Fig. 2b), are required for a complete characterization of the cross-bispectrum. For comparison, the bispectrumF(3)(ω1,ω2) fromFigure 2ais shown as a semi-transparent surface above the cross-bispectrum. (b) Bispectrum and cross-bispectrum along the lineω2=0, where they coincide. (c) Bispectrum (full blue line) and cross-bispectrum (dashed red line) along the lineω1=0. Higher order cross-correlations In Figure 3a , we finally consider the cross-bispectrum , measuring the third-order correlations between tunnelling electrons entering and leaving the SET. The three non-redundant permutations of the left and right pulse currents lead to a reduced symmetry of the cross-bispectrum, as visualized in comparison with the auto-correlation bispectrum in Figure 3a . The cross-bispectrum coincides with the auto-bispectrum on the line ω 2 =0, where they approach the zero-frequency correlation of the shot noise for ( Fig. 3b ). In contrast, for | ω 2 |≠0, the cross-bispectrum shows a frequency dependence similar to the cross-correlation shot noise and the anti-correlations due to the detection process become visible ( Fig. 3c ). Figure 3: Finite-frequency cross-bispectrum. ( a ) Measurements of the frequency-dependent cross-bispectrum . The cross-bispectrum shows a reduced symmetry compared with the bispectrum and measurements in the regions 1–3 ( Fig. 2b ), are required for a complete characterization of the cross-bispectrum. For comparison, the bispectrum F (3) ( ω 1 , ω 2 ) from Figure 2a is shown as a semi-transparent surface above the cross-bispectrum. ( b ) Bispectrum and cross-bispectrum along the line ω 2 =0, where they coincide. ( c ) Bispectrum (full blue line) and cross-bispectrum (dashed red line) along the line ω 1 =0. Full size image We have measured the current statistics of charge transport in an SET and directly determined the dynamical features and timescales of the current fluctuations. From the measured frequency-dependent noise power, we extracted the correlation time of the fluctuations. The noise power is a single-frequency quantity only, and to investigate the correlations between different spectral components of the current using bispectral analysis, we measured the frequency-dependent third order correlation function (the skewness). The skewness shows that the current statistics are non-gaussian on all frequencies owing to the applied voltage bias. Our experimental results are supported by model calculations that are in excellent agreement with measurements. The results presented here are important for future applications of SETs in nanoscale electrical circuits operating with single electrons. Our accurate and stable experiment also facilitates several promising directions for basic research on nanoscale quantum devices. These include experimental investigations of fluctuation relations at finite frequencies and higher order noise detection of interaction [42] and coherence-induced correlation effects [43] in quantum transport under non-equilibrium conditions. Device fabrication The device was fabricated by local anodic oxidation techniques using an atomic force microscope on the surface of a GaAs/AlGaAs heterostructure with electron density 4. 6×10 15 m −2 and a mobility of 64 m 2 /Vs. The two-dimensional electron gas residing 34 nm below the heterostructure surface is depleted underneath the oxidized lines, allowing us to define the QD and the QPC. Measurements The experiment was carried out in a 3 He cryostat at 500 mK with an applied bias of 900 μV across the QD to ensure unidirectional transport and to avoid the influence of thermal fluctuations. The QPC detector was tuned to the edge of the first conduction step. The current through the QPC was measured with a sampling frequency of 500 kHz. The tunnelling events were extracted from the QPC current using a step detection algorithm and converted into time-dependent pulse currents: Time was discretized in steps of Δ t =40 μs and in each step the number of tunnelling events Δ n in (out) of the QD was recorded. The current into (out of) the QD at a given time step is then I ( t )=(− e )Δ n/ Δ t . Error estimates We estimated the errors of the measured spectra by dividing the experimental data into 30 separate batches. The spectra were determined for each batch individually and their standard deviation was used as a measure of the experimental accuracy. Finite-frequency cumulants To define the finite-frequency cumulants of the current, we consider the m -time probability distribution [32] , [33] P ( m ) ( n 1 , t 1 ;...; n m , t m ) that n k electrons have been transferred during the time span [0, t k ] for k =1,..., m . The corresponding cumulant generating function is with χ =( χ 1 ,..., χ m ), t =( t 1 ,..., t m ), and n =( n 1 ,..., n m ). (An equivalent definition uses only a single but time-dependent counting field [44] .) The m -time cumulants of P ( m ) ( n ; t ) are then with the corresponding m -time cumulants of the current These equations define the cumulant averages denoted by double brackets . In the Fourier domain, the current cumulants can be expressed as as the sum of frequencies is zero in the stationary state. The Fourier-transformed current is denoted as and S ( m ) ( ω 1 , ω 2 ,..., ω m −1 ) is the polyspectrum [40] , which for m =2 and m =3 yields the noise spectrum S (2) ( ω ) (second cumulant) and the bispectrum (third cumulant) S (3) ( ω 1 , ω 2 ), respectively. We note that the noise spectrum S (2) ( ω ) in the stationary state is a single-frequency quantity that can be related directly to the one-time probability distribution P (1) ( n , t ) according to MacDonald's formula [45] The bispectrum F (3) ( ω 1 , ω 2 ) in contrast is a two-frequency quantity that reflects correlations of the current beyond what is captured by P (1) ( n , t ) alone. Theoretical model We consider the probability vector | p ( t )〉=[ p 00 ( t ), p 10 ( t ), p 01 ( t ), p 11 ( t )] T , where the first index denotes the number of (extra) electrons on the QD, i =0, 1, and the second index denotes the detected number of (extra) electrons on the QD as inferred from the current through the QPC, j =0, 1. The probability vector evolves according to the rate equation having introduced separate counting fields χ L and χ R that couple to the number of detected electrons that have passed the left and the right barriers, respectively [44] . The matrix M ( χ L , χ R ) reads [13] , [14] , [37] where factors of in the off-diagonal elements correspond to processes that increase by one the number of detected electrons that have tunnelled across the left (right) barrier ( Fig. 1c,d) . The detector rate Γ D of the QPC detector scheme tends to infinite for an ideal detector only, but is finite otherwise. Calculations For the calculations of the finite-frequency cumulants it is useful to write the matrix as where M 0 = M (0, 0) and I L(R) is the super operator for the detected current through the left (right) barrier [46] . Additionally, we need the stationary state , found by solving and normalized such that , where . We define the projectors [46] and Q = 1 − P and the frequency-dependent pseudoinverse [47] R ( ω )= Q [i ω + M 0 ] −1 Q , which is well-defined even in the zero-frequency limit ω →0, since the inversion is performed only in the subspace spanned by Q , where M 0 is regular. These objects constitute the essential building blocks for our calculations. The frequency-dependent second and third cumulants, S (2) ( ω ) and S (3) ( ω 1 , ω 2 ), can then be evaluated following refs 47 , 48 and 33 , respectively. How to cite this article: Ubbelohde, N. et al . Measurement of finite-frequency current statistics in a single-electron transistor. Nat. Commun. 3:612 doi: 10.1038/ncomms1620 (2012).